A fatty acid-dependent hypothalamic–DVC neurocircuitry that regulates hepatic secretion of triglyceride-rich lipoproteins The brain emerges as a regulator of hepatic triglyceride-rich very-low-density lipoproteins (VLDL-TG). The neurocircuitry involved as well as the ability of fatty acids to trigger a neuronal network to regulate VLDL-TG remain unknown. Here we demonstrate that infusion of oleic acid into the mediobasal hypothalamus (MBH) activates a MBH PKC-δ→K ATP -channel signalling axis to suppress VLDL-TG secretion in rats. Both NMDA receptor-mediated transmissions in the dorsal vagal complex (DVC) and hepatic innervation are required for lowering VLDL-TG, illustrating a MBH-DVC-hepatic vagal neurocircuitry that mediates MBH fatty acid sensing. High-fat diet (HFD)-feeding elevates plasma TG and VLDL-TG secretion and abolishes MBH oleic acid sensing to lower VLDL-TG. Importantly, HFD-induced dysregulation is restored with direct activation of either MBH PKC-δ or K ATP -channels via the hepatic vagus. Thus, targeting a fatty acid sensing-dependent hypothalamic–DVC neurocircuitry may have therapeutic potential to lower hepatic VLDL-TG and restore lipid homeostasis in obesity and diabetes. The metabolic syndrome includes atherogenic dyslipidemia that is due partly to an overproduction of triglyceride-rich very-low-density lipoproteins (VLDL-TG) by the liver and hypertriglyceridemia [1] , [2] . This disruption in lipid homeostasis also manifests in obesity and diabetes [3] , [4] . Given the impact of the morbidities associated with these conditions, there is a global effort to elucidate mechanisms underlying the regulation of lipid homeostasis in health and disease. Hormones and nutrients regulate whole-body lipid homeostasis. For example, catecholamines [5] , glucocorticoids [6] and insulin [5] as well as fatty acids and/or PPARγ activation [7] regulate adipocyte lipid metabolism. The liver maintains lipid homeostasis via its role in lipoprotein assembly and secretion as well as fatty acid synthesis and oxidation [8] , [9] . Leptin [10] , [11] and adiponectin [12] lower hepatic lipids in rodents, while insulin suppresses hepatic VLDL-TG secretion [13] , [14] . In contrast, fatty acids directly increase hepatic VLDL-TG secretion [15] , while glucose stimulates hepatic lipogenesis [16] , [17] . These studies indicate that hormone cues, and specifically lipids themselves, alter lipid metabolism in adipose tissue and liver. In addition, a contribution by the central nervous system (CNS) to overall lipid balance is becoming apparent. Centrally acting insulin [18] , ghrelin [19] , melanocortins [20] and leptin [21] , [22] alter lipid metabolism in adipose tissues and liver. Hypothalamic neuropeptide Y infusion augments VLDL-TG secretion [23] , [24] and impairs the ability of insulin to inhibit VLDL-TG secretion [25] . In contrast, glucose sensing in the mediobasal hypothalamus (MBH) [26] and glycine in the dorsal vagal complex (DVC) [27] suppress hepatic secretion of VLDL-TG. To date, the neurocircuitry involved in the central control of lipid homeostasis, as well as the ability of fatty acids to trigger a negative-feedback neuronal network to regulate hepatic VLDL-TG secretion, remain largely unknown. The potential for a MBH fatty acid-dependent neuronal network that regulates hepatic VLDL-TG secretion ( Fig. 1a ) stems from evidence that the hypothalamus senses fatty acids to lower appetite and glucose production [28] , [29] . Specifically, central oleic acid infusion inhibits food intake and glucose production [28] via shared mechanisms that mediate glucose sensing [30] . An increased level of oleic acid in the cerebrospinal fluid associates with improved glucose tolerance in humans [31] . Given that hypothalamic hormone signalling regulates hepatic lipid metabolism while fatty acid sensing regulates feeding and glucose production, we tested whether oleic acid infusion into the MBH regulates hepatic secretion of VLDL-TG in normal and high-fat diet (HFD)-induced hypertriglyceridemic rodents and characterized the associated MBH-sensing mechanisms and neurocircuitry ( Fig. 1a ). Here we show that MBH oleic acid sensory mechanisms trigger a MBH-DVC-hepatic vagal neuronal relay to regulate hepatic VLDL-TG secretion in vivo . 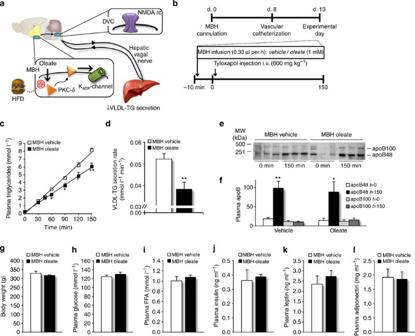Figure 1: MBH oleic acid and VLDL-TG secretion. (a) Schematic representation of working hypothesis: oleic acid triggers the translocation and activation of PKC-δ and subsequent activation of KATP-channels in the MBH, which activates a neuronal circuit involving NMDA receptors in the DVC and the hepatic vagal nerve, and lowers hepatic VLDL-TG secretion. HFD disrupts MBH oleic acid sensing to regulate VLDL-TG secretion. (b) Experimental protocol for experiments shown (c–l). MBH infusions of vehicle (white open squares,n=6) or oleic acid (black squares;n=8) were commenced att=−10 min after plasma samples were obtained. Time 0 min plasma samples were obtained after 10 min of MBH infusion, followed by an intravenous injection of tyloxapol (600 mg kg−1). Plasma samples were subsequently obtained every 15 min for the first hour and every 30 min until the end of the experiment att=150 min. (c) Plasma TG concentrations, (d) rates of appearance of VLDL-TG in plasma (*P<0.05; **P<0.006 versus vehicle infusion), (e) representative western blots and (f) protein levels of plasma apoB48 and apoB100 (in arbitrary units) following tyloxapol administration with MBH infusion of vehicle or oleic acid (*P<0.03; **P<0.002 versus apoB48t=0). (g) Body weights on the morning of tyloxapol experiments. Plasma (h) glucose, (i) FFA, (j) insulin, (k) leptin and (l) adiponectin concentrations att=150 min. Data are presented as mean+s.e.m. Unpaired, two-tailedt-tests were used for the statistical analyses of two groups. For measurements over time, repeated measures analysis of variance was used followed by Duncan’spost hoctest. Figure 1: MBH oleic acid and VLDL-TG secretion. ( a ) Schematic representation of working hypothesis: oleic acid triggers the translocation and activation of PKC-δ and subsequent activation of K ATP -channels in the MBH, which activates a neuronal circuit involving NMDA receptors in the DVC and the hepatic vagal nerve, and lowers hepatic VLDL-TG secretion. HFD disrupts MBH oleic acid sensing to regulate VLDL-TG secretion. ( b ) Experimental protocol for experiments shown ( c – l ). MBH infusions of vehicle (white open squares, n =6) or oleic acid (black squares; n =8) were commenced at t =−10 min after plasma samples were obtained. Time 0 min plasma samples were obtained after 10 min of MBH infusion, followed by an intravenous injection of tyloxapol (600 mg kg −1 ). Plasma samples were subsequently obtained every 15 min for the first hour and every 30 min until the end of the experiment at t =150 min. ( c ) Plasma TG concentrations, ( d ) rates of appearance of VLDL-TG in plasma (* P <0.05; ** P <0.006 versus vehicle infusion), ( e ) representative western blots and ( f ) protein levels of plasma apoB48 and apoB100 (in arbitrary units) following tyloxapol administration with MBH infusion of vehicle or oleic acid (* P <0.03; ** P <0.002 versus apoB48 t =0). ( g ) Body weights on the morning of tyloxapol experiments. Plasma ( h ) glucose, ( i ) FFA, ( j ) insulin, ( k ) leptin and ( l ) adiponectin concentrations at t =150 min. Data are presented as mean+s.e.m. Unpaired, two-tailed t -tests were used for the statistical analyses of two groups. For measurements over time, repeated measures analysis of variance was used followed by Duncan’s post hoc test. Full size image MBH oleic acid infusion lowers VLDL-TG secretion To evaluate whether MBH oleic acid sensing regulates VLDL-TG secretion in vivo , we first infused oleic acid directly into the MBH of 10-h fasted, freely moving, conscious, healthy rats ( Fig. 1b ). The secretion rate of VLDL-TG was determined as the rise in plasma TG levels over a 150-min period following intravenous tyloxapol (inhibitor of lipoprotein lipase) infusion. This 10-h fasting protocol yielded basal free fatty acid (FFA) levels of 0.61±0.04 and was chosen to minimize the contribution of intestinal chylomicrons. In rats fasted for as little as 4 h, chylomicrons were barely detectable compared with fed rats [23] , which suggest that chylomicrons do not contribute to the changes in VLDL-TG observed in the present study. In fact, no differences in the VLDL-TG secretion rates of rats fasted for 10 or 5 h were observed ( Supplementary Fig. 1 ). We discovered that MBH oleic acid infusion rapidly diminished the rise of plasma TG levels ( Fig. 1c ), which corresponded to an attenuated rate of VLDL-TG secretion ( Fig. 1d ) and was independent of differences in the increase of plasma apoB48 levels ( Fig. 1e,f ) and in body weight ( Fig. 1g ). Whereas plasma apoB48 levels increased in response to tyloxapol administration, there were no changes in plasma apoB100 levels, suggesting that apoB48, the predominant form of apoB lipoprotein in the rat liver [32] , but not apoB100 contributes to the rise in plasma VLDL-TG observed. In this regard, and since the intestinal contribution of chylomicrons is unlikely, the tyloxapol-induced rise in plasma TG measured is expected to correspond to changes to VLDL. This is supported by previous studies that investigated the role of the brain in the modulation of tyloxapol-induced TG secretion and characterized changes in TG levels to be part of fractions that contain VLDL (and not low-density lipoprotein (LDL) or high-density lipoprotein (HDL)) [23] , [26] , although analysis under the current experimental conditions warrants future analysis. We measured the plasma levels of nutrients and hormones at the final time point (150 min) and found that glucose ( Fig. 1h ), FFAs ( Fig. 1i ), insulin ( Fig. 1j ), leptin ( Fig. 1k ), adiponectin ( Fig. 1l ) were unchanged by MBH oleic acid infusion. Thus, MBH oleic acid sensing lowers VLDL-TG secretion independently of changes in circulating lipid-regulatory hormones and nutrients. Also, we found that MBH oleic acid versus vehicle infusion did not significantly alter HDL cholesterol and LDL/VLDL cholesterol levels (150 min, Supplementary Fig. 2a,b ) but increase plasma total bile acid levels (150 min, Supplementary Fig. 2c ), which warrants future investigation. MBH PKC-δ and hepatic scd-1 mediate MBH oleic acid’s effect To explore downstream MBH fatty acid-dependent mechanisms, we evaluated the role of MBH PKC-δ ( Fig. 2a,b ). MBH PKC-δ was first tested since the activation of MBH PKC-δ is necessary for lipids to lower glucose production [33] and glucagon-like peptide 1 to regulate insulin sensitivity [34] . Further, oleic acid directly activates PKC-δ in hepatocytes [35] . 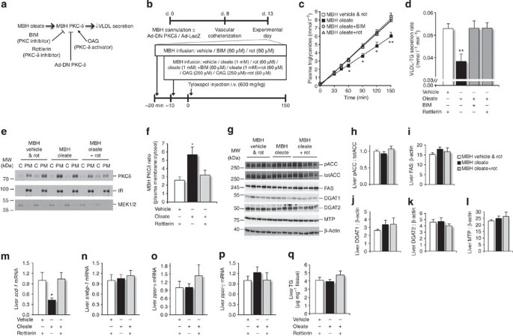Figure 2: MBH oleic acid-PKC-δ activation and hepaticscd-1mRNA expression. (a) Schematic representation of working hypothesis. (b) Experimental protocol for experiments shown (c,d) andFig. 3a–d: MBH preinfusions of vehicle, bisindolylmaleimide (BIM) or rottlerin (rot) were commenced at −20 min, and infusions of vehicle, oleic acid, oleic acid+BIM, oleic acid+rot, 1-OAG or OAG+rot were commenced att=−10 min. (c) Plasma TG concentrations and (d) rates of appearance of VLDL-TG in plasma with MBH infusion of vehicle and rot (white squares,n=7), oleic acid (black squares,n=8), oleic acid+BIM (grey circles,n=7) or oleic acid+rot (grey triangles,n=6). *P<0.04, **P<0.007 oleic acid versus other groups. (e) Representative western blots of PKC-δ (top), IR and mitogen-activated protein kinase 1/2 (MEK1/2) protein levels in cytosolic (C) and plasma membrane (PM) fractions in and (f) ratios of plasma membrane PKC-δ: cytosolic PKC-δ protein concentrations of, MBH tissues treated with vehicle and rot (n=8), oleic acid (n=7) or oleic acid+rot (n=8). *P<0.05 versus other groups. MW, molecular weight. (g) Representative western blots and ratios of protein levels of (h) phosphorylated acetyl-CoA carboxylase (pACC) to total acetyl-CoA carboxylase (totACC) and (i) FAS, (j) diacylglycerol acyltransferase 1 (DGAT1), (k) diacylglycerol acyltransferase 2 (DGAT2) and (l) microsomal MTP to β-actin in livers from experiments shown inc,d. Expressions of mRNA (fold-increase versus vehicle and rot) of (m) stearoyl-CoA desaturase (scd-1), (n) sterol regulatory element-binding protein 1 (srebp-1), (o) peroxisome proliferator-activated receptor α (ppar-α) and (p) peroxisome proliferator-activated receptor γ (ppar-γ) in livers from experiments shown inc,d. *P<0.05 versus other groups. (q) TG content in livers from experiments shown inc,d. Data are presented as mean+s.e.m. Statistical significance determined by Dunnett’spost hoctest after analysis of variance (ANOVA). For measurements over time, repeated measures ANOVA was used followed by Duncan’spost hoctest. Figure 2: MBH oleic acid-PKC-δ activation and hepatic scd-1 mRNA expression. ( a ) Schematic representation of working hypothesis. ( b ) Experimental protocol for experiments shown ( c , d ) and Fig. 3a–d : MBH preinfusions of vehicle, bisindolylmaleimide (BIM) or rottlerin (rot) were commenced at −20 min, and infusions of vehicle, oleic acid, oleic acid+BIM, oleic acid+rot, 1-OAG or OAG+rot were commenced at t =−10 min. ( c ) Plasma TG concentrations and ( d ) rates of appearance of VLDL-TG in plasma with MBH infusion of vehicle and rot (white squares, n =7), oleic acid (black squares, n =8), oleic acid+BIM (grey circles, n =7) or oleic acid+rot (grey triangles, n =6). * P <0.04, ** P <0.007 oleic acid versus other groups. ( e ) Representative western blots of PKC-δ (top), IR and mitogen-activated protein kinase 1/2 (MEK1/2) protein levels in cytosolic (C) and plasma membrane (PM) fractions in and ( f ) ratios of plasma membrane PKC-δ: cytosolic PKC-δ protein concentrations of, MBH tissues treated with vehicle and rot ( n =8), oleic acid ( n =7) or oleic acid+rot ( n =8). * P <0.05 versus other groups. MW, molecular weight. ( g ) Representative western blots and ratios of protein levels of ( h ) phosphorylated acetyl-CoA carboxylase (pACC) to total acetyl-CoA carboxylase (totACC) and ( i ) FAS, ( j ) diacylglycerol acyltransferase 1 (DGAT1), ( k ) diacylglycerol acyltransferase 2 (DGAT2) and ( l ) microsomal MTP to β-actin in livers from experiments shown in c , d . Expressions of mRNA (fold-increase versus vehicle and rot) of ( m ) stearoyl-CoA desaturase (scd-1), ( n ) sterol regulatory element-binding protein 1 (srebp-1), ( o ) peroxisome proliferator-activated receptor α (ppar-α) and ( p ) peroxisome proliferator-activated receptor γ (ppar-γ) in livers from experiments shown in c , d . * P <0.05 versus other groups. ( q ) TG content in livers from experiments shown in c , d . Data are presented as mean+s.e.m. Statistical significance determined by Dunnett’s post hoc test after analysis of variance (ANOVA). For measurements over time, repeated measures ANOVA was used followed by Duncan’s post hoc test. Full size image We discovered that concurrent MBH infusion of a general PKC inhibitor bisindolylmaleimide (BIM), or of a specific PKC-δ inhibitor rottlerin, nullified the ability of MBH oleic acid to lower plasma TG and VLDL-TG secretion ( Fig. 2c,d ). We further measured the relative quantities of PKC-δ protein in purified plasma membrane (confirmed with the exclusive presence of insulin receptor (IR; Fig. 2e )) and cytosolic fractions (confirmed with the marked enrichment of MEK1/2 ( Fig. 2e )) of MBH tissue treated with oleic acid. The translocation of PKC-δ from the cytosol to the plasma membrane, an indication of its activity [36] , [37] , was increased 2-fold by oleic acid infusion in MBH tissue as compared with vehicle infusion ( Fig. 2e,f ). Importantly, PKC-δ inhibition with rottlerin at the same dose that blocked the hypolipidemic effect of oleic acid ( Fig. 2c,d ) reversed the oleic acid-induced enrichment of PKC-δ in the plasma membrane ( Fig. 2e,f ). To delineate the hepatic mechanisms, protein levels of lipogenic biomarkers were measured in livers immediately obtained following infusion studies ( Fig. 2g ). The hypolipidemic effect of MBH oleic acids, and its reversal with MBH PKC-δ inhibition, occurred independently of changes in hepatic levels of acetyl-CoA carboxylase (ACC), fatty acid synthase (FAS), diacylglycerol acyltransferase 1 (DGAT1), diacylglycerol acyltransferase 2 (DGAT2) and microsomal triglyceride transfer protein (MTP; Fig. 2h–l ). We further assessed the expression of hepatic genes relevant to de novo lipogenesis and triglyceride metabolism. Importantly, hepatic stearoyl-CoA desaturase ( scd-1 ) expression was reduced with MBH oleic acid infusion, and this change was reversed with MBH PKC-δ inhibition ( Fig. 2m ). However, the hepatic mRNA expressions of sterol regulatory element-binding protein 1 ( srebp-1 ) and peroxisome proliferator-activated receptor-α and -γ ( ppar-α and ppar-γ ) were unchanged ( Fig. 2n–p ). Furthermore, MBH oleic acid infusion did not affect hepatic TG content ( Fig. 2q ). Together this suggests that MBH oleic acid activates PKC-δ and suppresses VLDL-TG secretion via an inhibition of hepatic scd-1 independent of changes in hepatic TG synthesis. To alternatively inhibit MBH PKC-δ, we injected an adenovirus expressing the dominant negative (DN) form of PKC-δ, or LacZ as a control, directly into the MBH ( Fig. 2a,b ). Notably, this DN form of PKC-δ carries a mutation in the catalytic region of the enzyme that abolishes its ATP-binding ability [38] , and the injection of DN PKC-δ was previously demonstrated to elicit a ~60% reduction in tissue PKC-δ activity [39] . We here confirmed that direct injection of DN PKC-δ into the MBH of rats selectively increased PKC-δ, but not another relevant isoform such as PKC-ε, in the MBH ( Supplementary Fig. 3 ). MBH vehicle infusion in rats injected with either of the adenoviruses yielded similar plasma lipid profiles ( Fig. 3a,b ) as those without adenovirus ( Fig. 1c,d ). MBH oleic acid failed to lower plasma TG and VLDL-TG secretion in rats injected with the DN PKC-δ as compared with LacZ ( Fig. 3a,b ). Collectively, both molecular and chemical loss-of-function experiments demonstrate that MBH oleic acid activates PKC-δ to lower VLDL-TG secretion ( Fig. 1a ). 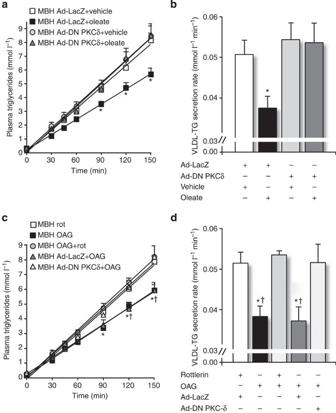Figure 3: MBH PKC-δ activation and VLDL-TG secretion. Experimental protocol shown inFig. 2b. Independent groups received adenoviral injection of LacZ or DN PKC-δ immediately following stereotaxic surgery as indicated. (a) Plasma TG concentrations and (b) rates of appearance of VLDL-TG in plasma in rats with prior adenoviral LacZ injection with MBH infusion of vehicle (white open squares,n=5) or oleic acid (black squares,n=6) or adenoviral DN PKC-δ injection with MBH infusion of vehicle (grey circles,n=6 or oleic acid (grey triangles,n=6). *P<0.05 versus other groups. (c) Plasma TG concentrations and (d) rates of appearance of VLDL-TG in plasma with MBH infusion of rot (white open squares,n=5), OAG (black squares,n=5), OAG+rot (grey circles,n=6) and in rats with prior adenoviral LacZ injection with OAG (dark grey triangles,n=7) or adenoviral DN PKC-δ injection with OAG (light grey triangles,n=5). *P<0.01 OAG versus rot, OAG+rot; †P<0.05 LacZ+OAG versus DN PKC-δ+OAG. Data are presented as mean+s.e.m. Statistical significance determined by Dunnett’spost hoctest after analysis of variance (ANOVA). For measurements over time, repeated measures ANOVA was used followed by Duncan’spost hoctest. Figure 3: MBH PKC-δ activation and VLDL-TG secretion. Experimental protocol shown in Fig. 2b . Independent groups received adenoviral injection of LacZ or DN PKC-δ immediately following stereotaxic surgery as indicated. ( a ) Plasma TG concentrations and ( b ) rates of appearance of VLDL-TG in plasma in rats with prior adenoviral LacZ injection with MBH infusion of vehicle (white open squares, n =5) or oleic acid (black squares, n =6) or adenoviral DN PKC-δ injection with MBH infusion of vehicle (grey circles, n =6 or oleic acid (grey triangles, n =6). * P <0.05 versus other groups. ( c ) Plasma TG concentrations and ( d ) rates of appearance of VLDL-TG in plasma with MBH infusion of rot (white open squares, n =5), OAG (black squares, n =5), OAG+rot (grey circles, n =6) and in rats with prior adenoviral LacZ injection with OAG (dark grey triangles, n =7) or adenoviral DN PKC-δ injection with OAG (light grey triangles, n =5). * P <0.01 OAG versus rot, OAG+rot; † P <0.05 LacZ+OAG versus DN PKC-δ+OAG. Data are presented as mean+s.e.m. Statistical significance determined by Dunnett’s post hoc test after analysis of variance (ANOVA). For measurements over time, repeated measures ANOVA was used followed by Duncan’s post hoc test. Full size image MBH PKC-δ activation lowers VLDL-TG secretion To address whether MBH PKC-δ activation is sufficient to lower VLDL-TG secretion, we infused PKC activator 1-oleoyl-2-acetyl- sn -glycerol (OAG) into the MBH and monitored plasma TG levels as above ( Fig. 3c,d ). MBH OAG infusion as compared with rottlerin alone (i) lowered plasma TG and VLDL-TG secretion to a similar extent as MBH oleic acid ( Figs 2c,d and 3c,d ) and (ii) induced MBH PKC-δ translocation by twofold (PKC-δ plasma membrane:cytosol ratios 3.6±0.4 (rottlerin alone, n =11) versus 7.2±0.7 (OAG, n =11); P <0.001, analysis of variance (ANOVA), followed by Dunnett’s post hoc test). Concurrent MBH rottlerin infusion with OAG nullified the ability of OAG to lower VLDL-TG secretion ( Fig. 3c,d ) and induce PKC-δ translocation (PKC-δ plasma membrane:cytosol ratio 4.0±0.7 (OAG+rottlerin, n =6)). We repeated MBH OAG infusion experiments in rats that received either MBH LacZ or DN PKC-δ injection and found that MBH OAG failed to lower plasma TG and VLDL-TG secretion in MBH DN PKC-δ as compared with LacZ-injected rats ( Fig. 3c,d ). Thus, direct MBH PKC-δ activation is sufficient to recapitulate the hypolipidemic effect of MBH oleic acid. MBH K ATP -channel activation lowers VLDL-TG secretion Given that the activation of MBH K ATP -channels is necessary for lipid-PKC activation to lower glucose production [33] , we addressed the role of MBH K ATP -channels in the VLDL-TG lowering effect of MBH oleic acid→PKC-δ signalling via chemical and molecular loss-of-function approaches ( Fig. 4a,b ). MBH infusion of K ATP -channel inhibitor glibenclamide negated the effect of oleic acid to suppress plasma TG and VLDL-TG ( Fig. 4c,d ), independently of changes in plasma insulin levels ( Fig. 4e ). K ATP -channels sensitive to glibenclamide, comprised of SUR1 receptor proteins and Kir6.2 pore-forming subunits, are found in β-cells of the pancreas and in neurons [40] . Thus, we next injected an adenovirus expressing a DN form of the Kir6.2 subunit (or green fluorescent protein (GFP) as a control) into the MBH to inhibit K ATP -channel activity. This construct, consisting of a 3-amino substitution in the selectivity filter, co-assembles with nascent Kir6.2 but prevents potassium conductance [41] . MBH oleic acid infusion lowered plasma TG and VLDL-TG secretion in GFP-control virus treated rats but failed to suppress plasma TG and VLDL-TG in rats expressing mutant MBH K ATP -channels ( Fig. 4f,g ). To confirm that MBH PKC-δ signals between oleic acid and K ATP -channels ( Fig. 4a ), we repeated the MBH K ATP -channel targeted inhibitory experiments with OAG infusion. Whereas MBH OAG lowered lipids in GFP-control rats, its effect was nullified in rats lacking functional MBH K ATP -channels ( Fig. 4f,g ). 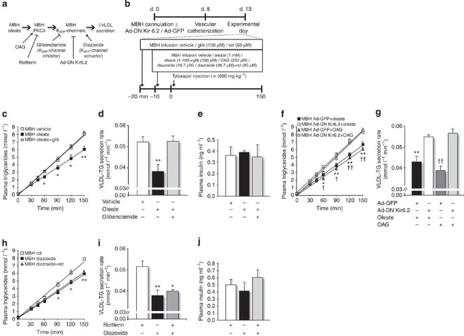Figure 4: MBH KATP-channel activation and VLDL-TG secretion. (a) Schematic representation of working hypothesis. (b) Experimental protocol: independent rats received adenoviral injection of GFP or DN Kir6.2 immediately following stereotaxic surgery as indicated (f,g). MBH preinfusions of vehicle, glibenclamide (glib) or rot were commenced at −20 min, and infusions of vehicle, oleic acid, oleic acid+glib, OAG, diazoxide or diazoxide+rot were commenced att=−10 min. (c) TG concentrations, (d) rates of appearance of VLDL-TG and (e) insulin concentrations in plasma with MBH infusion of vehicle (white open squares,n=6), oleic acid (black squares,n=8) or oleic acid+glib (grey circles,n=5). *P<0.04; **P<0.008 versus other groups. (f) Plasma TG concentrations and (g) rates of appearance of VLDL-TG in plasma in rats with prior adenoviral GFP injection following MBH infusion of oleic acid (black squares,n=7) or OAG (grey triangles,n=4) or adenoviral DN Kir6.2 injection with oleic acid (white open squares,n=4) or OAG (grey circles,n=5). *P<0.03, **P<0.001 GFP+oleic acid versus DN Kir6.2+oleic acid. †P<0.03, ††P<0.004 GFP+OAG versus DN Kir6.2+OAG. (h) TG concentrations, (i) rates of appearance of VLDL-TG and (j) insulin concentrations in plasma following MBH infusion of rot (white open squares,n=5), diazoxide (black squares,n=6) or diazoxide+rot (grey triangles,n=6). *P<0.04; **P<0.009 diazoxide, diazoxide+rot versus rot. Data are presented as mean+s.e.m. Statistical significance determined by Dunnett’spost hoctest after analysis of variance (ANOVA). For measurements over time, repeated measures ANOVA was used followed by Duncan’spost hoctest. Figure 4: MBH K ATP -channel activation and VLDL-TG secretion. ( a ) Schematic representation of working hypothesis. ( b ) Experimental protocol: independent rats received adenoviral injection of GFP or DN Kir6.2 immediately following stereotaxic surgery as indicated ( f , g ). MBH preinfusions of vehicle, glibenclamide (glib) or rot were commenced at −20 min, and infusions of vehicle, oleic acid, oleic acid+glib, OAG, diazoxide or diazoxide+rot were commenced at t =−10 min. ( c ) TG concentrations, ( d ) rates of appearance of VLDL-TG and ( e ) insulin concentrations in plasma with MBH infusion of vehicle (white open squares, n =6), oleic acid (black squares, n =8) or oleic acid+glib (grey circles, n =5). * P <0.04; ** P <0.008 versus other groups. ( f ) Plasma TG concentrations and ( g ) rates of appearance of VLDL-TG in plasma in rats with prior adenoviral GFP injection following MBH infusion of oleic acid (black squares, n =7) or OAG (grey triangles, n =4) or adenoviral DN Kir6.2 injection with oleic acid (white open squares, n =4) or OAG (grey circles, n =5). * P <0.03, ** P <0.001 GFP+oleic acid versus DN Kir6.2+oleic acid. † P <0.03, †† P <0.004 GFP+OAG versus DN Kir6.2+OAG. ( h ) TG concentrations, ( i ) rates of appearance of VLDL-TG and ( j ) insulin concentrations in plasma following MBH infusion of rot (white open squares, n =5), diazoxide (black squares, n =6) or diazoxide+rot (grey triangles, n =6). * P <0.04; ** P <0.009 diazoxide, diazoxide+rot versus rot. Data are presented as mean+s.e.m. Statistical significance determined by Dunnett’s post hoc test after analysis of variance (ANOVA). For measurements over time, repeated measures ANOVA was used followed by Duncan’s post hoc test. Full size image We next discovered that the direct infusion of K ATP -channel activator diazoxide into the MBH lowered plasma TG and VLDL-TG secretion ( Fig. 4h,i ), independently of changes in plasma insulin levels ( Fig. 4j ). Simultaneous MBH PKC-δ inactivation with rottlerin infusion did not reverse the lipid-lowering effect of MBH diazoxide ( Fig. 4h,i ), confirming that MBH K ATP -channel activation is downstream of MBH oleic acid→PKC-δ signalling. These data indicate that the activation of MBH K ATP -channels is sufficient and necessary for MBH oleic acid→PKC-δ signalling to lower VLDL-TG secretion ( Fig. 1a ). A MBH→DVC→hepatic vagal neurocircuitry regulates VLDL-TG N -methyl- D -aspartate (NMDA) receptor-mediated transmission in the DVC is sufficient and necessary for MBH nutrient sensing to lower glucose production [42] , [43] and is also sufficient to lower hepatic VLDL-TG secretion [27] . To begin delineating the neurocircuitry that mediates the lipid-lowering effect of MBH oleic acid sensing ( Fig. 1a ), we first implanted independent bilateral catheters into both the MBH and DVC of the same rats. This model enables the concurrent delivery of substances into the MBH and DVC independent of direct infusate contact and thus assesses the neuronal communication between MBH and DVC in vivo. On recovery, we repeated the VLDL-TG secretion monitoring in the presence of MBH oleic acid infusion and inhibition of DVC NMDA receptor-mediated transmission via NMDA receptor blocker MK-801 ( Fig. 5a ). Concurrent infusion of MK-801, but not saline, into the DVC abolished the lipid-lowering effect of MBH oleic acid infusion ( Fig. 5b,c ). 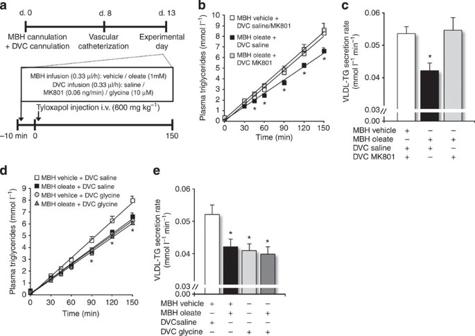Figure 5: MBH oleic acid and a DVC NMDA receptor-dependent mechanism. (a) Experimental protocol: stereotaxic placement of cannulae into both the MBH and DVC. DVC preinfusions of saline or MK-801 were commenced att=−20 min and simultaneous MBH infusions of vehicle or oleic acid were commenced att=−10 min. (b) Plasma TG concentrations and (c) rates of appearance of VLDL-TG in plasma following MBH infusion of vehicle and concurrent DVC infusion of saline or MK-801 (white open squares,n=10 comprised ofn=5 DVC saline andn=5 DVC MK-801) or MBH of oleic acid and concurrent DVC infusion of saline (black squares,n=7) or MK-801 (grey squares,n=7). *P<0.02; versus other groups. (d) Plasma TG concentrations and (e) rates of appearance of VLDL-TG in plasma following MBH infusion of vehicle and concurrent DVC infusion of saline (white open squares,n=5) or DVC glycine (grey circles,n=7) or MBH infusion of oleic acid with concurrent DVC infusion of saline (black squares,n=7) or DVC glycine (grey triangles,n=6). *P<0.05; versus MBH vehicle+DVC saline. Data are presented as mean+s.e.m. Statistical significance determined by Dunnett’spost hoctest after analysis of variance (ANOVA). For measurements over time, repeated measures ANOVA was used followed by Duncan’spost hoctest. Figure 5: MBH oleic acid and a DVC NMDA receptor-dependent mechanism. ( a ) Experimental protocol: stereotaxic placement of cannulae into both the MBH and DVC. DVC preinfusions of saline or MK-801 were commenced at t =−20 min and simultaneous MBH infusions of vehicle or oleic acid were commenced at t =−10 min. ( b ) Plasma TG concentrations and ( c ) rates of appearance of VLDL-TG in plasma following MBH infusion of vehicle and concurrent DVC infusion of saline or MK-801 (white open squares, n =10 comprised of n =5 DVC saline and n =5 DVC MK-801) or MBH of oleic acid and concurrent DVC infusion of saline (black squares, n =7) or MK-801 (grey squares, n =7). * P <0.02; versus other groups. ( d ) Plasma TG concentrations and ( e ) rates of appearance of VLDL-TG in plasma following MBH infusion of vehicle and concurrent DVC infusion of saline (white open squares, n =5) or DVC glycine (grey circles, n =7) or MBH infusion of oleic acid with concurrent DVC infusion of saline (black squares, n =7) or DVC glycine (grey triangles, n =6). * P <0.05; versus MBH vehicle+DVC saline. Data are presented as mean+s.e.m. Statistical significance determined by Dunnett’s post hoc test after analysis of variance (ANOVA). For measurements over time, repeated measures ANOVA was used followed by Duncan’s post hoc test. Full size image Given that glycine infusion into the DVC activates DVC NMDA receptors to lower VLDL-TG secretion [27] , we tested for a potential additive or redundant role of MBH oleic acid and DVC glycine to lower hepatic VLDL-TG secretion. The independent hypolipidemic effects of MBH oleic acid and DVC glycine infusions were not additive ( Fig. 5d,e ). Taken together, MBH oleic acid acts via a DVC NMDA receptor-dependent mechanism to suppress hepatic VLDL-TG secretion, and the brain has redundant nutrient-sensing mechanisms to regulate peripheral lipid homeostasis. We examined the effect of hepatic vagal denervation on MBH oleic acid infusion ( Fig. 6a ). The suppression of hypertriglyceridemia and hepatic VLDL-TG as observed with MBH oleic acid compared with vehicle infusion was abolished in rats that underwent hepatic vagotomy as compared with sham vagotomy ( Fig. 6b,c ), independently of changes in plasma glucose or FFA levels ( Fig. 6d,e ). Hepatic or sham vagotomy alone neither affected VLDL-TG secretion profiles within the current experimental conditions ( Fig. 6b,c ), nor plasma glucose or FFA levels ( Fig. 6d,e ). Taken together, MBH oleic acid triggers a MBH–DVC–hepatic vagal neurocircuitry to lower hepatic secretion of VLDL-TG. 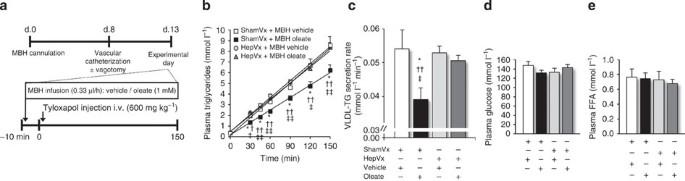Figure 6: MBH oleic acid and hepatic vagal innervation. (a) Experimental protocol: immediately preceding vascular catheterization, rats underwent a hepatic vagotomy (HepVx) or sham operation (ShamVx). MBH preinfusions of vehicle or oleic acid were commenced att=−10 min. (b) TG concentrations, (c) rates of appearance of VLDL-TG, (d) glucose concentrations and (e) FFA concentrations in plasma in sham-operated rats with MBH infusion of vehicle (white open squares,n=6) or oleic acid (black squares,n=7) or vagotomized rats with vehicle (grey circles,n=4) or oleic acid (grey triangles,n=6). *P<0.05 versus ShamVx+vehicle. †P<0.02, ††P<0.008 versus HepVx+vehicle. ‡P<0.02, ‡‡P<0.008 versus HepVx+oleic acid. Data are presented as mean+s.e.m. Statistical significance determined by Dunnett’spost hoctest after analysis of variance (ANOVA). For measurements over time, repeated measures ANOVA was used followed by Duncan’spost hoctest. Figure 6: MBH oleic acid and hepatic vagal innervation. ( a ) Experimental protocol: immediately preceding vascular catheterization, rats underwent a hepatic vagotomy (HepVx) or sham operation (ShamVx). MBH preinfusions of vehicle or oleic acid were commenced at t =−10 min. ( b ) TG concentrations, ( c ) rates of appearance of VLDL-TG, ( d ) glucose concentrations and ( e ) FFA concentrations in plasma in sham-operated rats with MBH infusion of vehicle (white open squares, n =6) or oleic acid (black squares, n =7) or vagotomized rats with vehicle (grey circles, n =4) or oleic acid (grey triangles, n =6). * P <0.05 versus ShamVx+vehicle. † P <0.02, †† P <0.008 versus HepVx+vehicle. ‡ P <0.02, ‡‡ P <0.008 versus HepVx+oleic acid. Data are presented as mean+s.e.m. Statistical significance determined by Dunnett’s post hoc test after analysis of variance (ANOVA). For measurements over time, repeated measures ANOVA was used followed by Duncan’s post hoc test. Full size image MBH oleic acid sensing in HFD-induced hypertriglyceridemia In a model of short-term HFD feeding in which hepatic VLDL-TG secretion and plasma TG levels are elevated [26] , [27] , [44] , we investigated whether MBH oleic acid sensing-dependent neurocircuitry is intact ( Fig. 7a ). 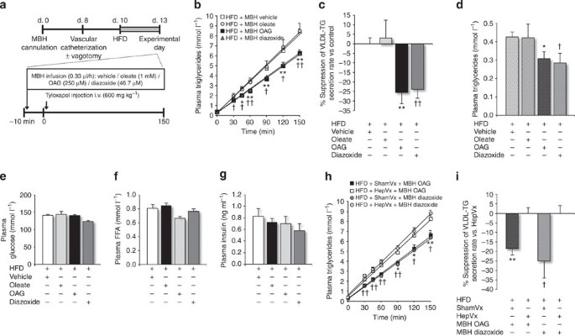Figure 7: MBH oleic acid sensory mechanisms in HFD-induced hypertriglyceridemia. (a) Experimental protocol: three days before the experimental day, rats were introduced to and maintained on a lard oil-enriched HFD. In a separate set of experiments shown (h,i), rats underwent a hepatic vagotomy (HepVx) or sham operation (ShamVx) immediately preceding vascular catheterization. MBH infusions of vehicle, oleic acid, OAG or diazoxide were commenced att=−10 min. (b) Plasma TG concentrations and (c) per cent suppression of VLDL-TG secretion rate as compared with control with MBH infusion of vehicle (white open squares,n=6), oleic acid (grey circles,n=5), OAG (black squares,n=6) or diazoxide (grey triangles,n=5). *P<0.04; **P<0.008 HFD+OAG versus HFD+vehicle. †P<0.02, ††P<0.007 HFD+diazoxide versus HFD+vehicle. Data are presented as mean+s.e.m. (d) Plasma TG in non-tyloxapol-treated rats given MBH infusions of vehicle (n=8), oleic acid (1 mM,n=6), OAG (250 μM,n=4) or diazoxide (46.7 μM,n=5). *P<0.05; **P<0.008 HFD+OAG versus HFD+vehicle. †P<0.05, ††P<0.007 HFD+diazoxide versus HFD+vehicle. Plasma (e) glucose, (f) FFA and (g) insulin concentrations in HFD-fed rats from experiments shown (b,c). (h) Plasma TG concentrations and (i) per cent suppression of VLDL-TG secretion rate as compared with respective HFD-fed HepVx controls in HFD-fed sham-operated rats with MBH infusion of OAG (black squares,n=8) or diazoxide (dark grey circles,n=6) or vagotomized rats with OAG (white squares,n=5), or diazoxide (light grey circles,n=5). *P<0.05; **P<0.004 HFD+ShamVx+OAG versus HFD+HepVx+OAG. †P<0.05, ††P<0.007 HFD+ShamVx+diazoxide versus HFD+HepVx+diazoxide. Data are presented as mean+s.e.m. Statistical significance determined by Dunnett’spost hoctest after analysis of variance (ANOVA). For measurements over time, repeated measures ANOVA was used followed by Duncan’spost hoctest. Figure 7: MBH oleic acid sensory mechanisms in HFD-induced hypertriglyceridemia. ( a ) Experimental protocol: three days before the experimental day, rats were introduced to and maintained on a lard oil-enriched HFD. In a separate set of experiments shown ( h , i ), rats underwent a hepatic vagotomy (HepVx) or sham operation (ShamVx) immediately preceding vascular catheterization. MBH infusions of vehicle, oleic acid, OAG or diazoxide were commenced at t =−10 min. ( b ) Plasma TG concentrations and ( c ) per cent suppression of VLDL-TG secretion rate as compared with control with MBH infusion of vehicle (white open squares, n =6), oleic acid (grey circles, n =5), OAG (black squares, n =6) or diazoxide (grey triangles, n =5). * P <0.04; ** P <0.008 HFD+OAG versus HFD+vehicle. † P <0.02, †† P <0.007 HFD+diazoxide versus HFD+vehicle. Data are presented as mean+s.e.m. ( d ) Plasma TG in non-tyloxapol-treated rats given MBH infusions of vehicle ( n =8), oleic acid (1 mM, n =6), OAG (250 μM, n =4) or diazoxide (46.7 μM, n =5). * P <0.05; ** P <0.008 HFD+OAG versus HFD+vehicle. † P <0.05, †† P <0.007 HFD+diazoxide versus HFD+vehicle. Plasma ( e ) glucose, ( f ) FFA and ( g ) insulin concentrations in HFD-fed rats from experiments shown ( b , c ). ( h ) Plasma TG concentrations and ( i ) per cent suppression of VLDL-TG secretion rate as compared with respective HFD-fed HepVx controls in HFD-fed sham-operated rats with MBH infusion of OAG (black squares, n =8) or diazoxide (dark grey circles, n =6) or vagotomized rats with OAG (white squares, n =5), or diazoxide (light grey circles, n =5). * P <0.05; ** P <0.004 HFD+ShamVx+OAG versus HFD+HepVx+OAG. † P <0.05, †† P <0.007 HFD+ShamVx+diazoxide versus HFD+HepVx+diazoxide. Data are presented as mean+s.e.m. Statistical significance determined by Dunnett’s post hoc test after analysis of variance (ANOVA). For measurements over time, repeated measures ANOVA was used followed by Duncan’s post hoc test. Full size image Three days of HFD feeding in rats elicited fasting (10 h) hypertriglyceridemia (plasma TG levels with regular chow: 0.32±0.02 mM versus HFD: 0.43±0.03 mM, P <0.05, t -test), mild fasting hyperglycaemia (plasma glucose levels with regular chow: 131.0±4.0 mg dl −1 versus HFD: 142.3±1.8 mg dl −1 , P <0.05, t -test), fasting hyperinsulinemia (plasma insulin levels with regular chow: 0.7±0.1 ng ml −1 versus HFD: 1.4±0.1 ng ml −1 , P <0.002, t -test), but no significant changes in fasting FFA levels (plasma FFA levels in rats fed with regular chow: 0.61±0.04 mM versus HFD: 0.51±0.06 mM). In addition, 3 days of high-fat feeding elicited a tyloxapol-induced hypersecretion of VLDL-TG by 26.3±9.8% as compared with regular chow-fed controls ( P <0.05, t -test). This disruption of lipid homeostasis was associated with the inability of MBH oleic acid as compared with vehicle infusion (i) to suppress hepatic VLDL-TG secretion rates in tyloxapol-treated HFD-fed rats ( Fig. 7b,c ) and (ii) to lower plasma TG levels in non-tyloxapol-treated HFD-fed rats ( Fig. 7d ). Importantly, direct activation of downstream signalling effectors ( Fig. 1a ) via MBH infusion of OAG or diazoxide bypassed this impairment of MBH oleic acid, lowering hepatic VLDL-TG secretion ( Fig. 7b,c ), independently of changes in plasma glucose, FFA or insulin levels ( Fig. 7e–g ) and plasma TG levels in HFD-fed rats ( Fig. 7d ). Hepatic-vagotomized (or sham-operated) rats that were fed with a HFD for 3 days underwent tyloxapol-induced VLDL-TG secretion experiments while receiving MBH OAG or MBH diazoxide infusions ( Fig. 7a ). Sham rats that were given MBH OAG or diazoxide had lower plasma TG and VLDL-TG secretion rates as compared with their vagotomized counterparts ( Fig. 7h,i ). Thus, HFD-induced hypertriglyceridemia and hypersecretion of VLDL-TG are associated with a disruption of MBH oleic acid sensing that normally restrains hepatic VLDL-TG secretion, and this disruption is circumvented by activating downstream mediators of the MBH oleic acid signalling pathway (that is, PKC-δ and K ATP -channels) via the hepatic vagus. The excessive consumption of lipogenic calories leads to dyslipidemia and ectopic lipid deposition in the tissues, giving rise to deleterious health consequences [45] . This disruption in lipid homeostasis induces insulin resistance in the brain [29] as well as the periphery [46] . Resistance to the suppressive effects of insulin augments hepatic VLDL-TG production [9] , further contributing to obesity-related lipidemic abnormalities. Our current discoveries highlight the role of the MBH that senses oleic acid to suppress the hepatic secretion of VLDL-TG and maintain lipid homeostasis. With molecular, chemical and surgical loss- and gain-of-function approaches, we demonstrate that this fatty acid-dependent neurocircuitry involves the activation of a MBH PKC-δ→K ATP -channel axis and DVC NMDA receptor-mediated neurotransmission to signal via the hepatic vagus to lower VLDL-TG. Of note, reduced MBH PKC-δ signalling per se does not disrupt VLDL secretion (but blocks the hypolipidemic effects of MBH oleic acid infusion), suggesting that the basal tone of the CNS–liver circuitry does not necessarily regulate VLDL secretion. Rather, we propose that the existing fatty acid-dependent brain–liver neurocircuitry plays a vital role to maintain lipid homeostasis in a post-prandial condition. MBH oleic acid-PKC-δ-induced reduction of VLDL-TG secretion associates with an inhibition of hepatic scd-1 mRNA expression, which is corroborated by previous CNS-hepatic lipid metabolic studies [21] , [23] , [26] , [27] , [47] , [48] , but is independent of changes in hepatic MTP levels and plasma apoB lipoprotein levels. Scd-1 catalyses the desaturation of saturated fatty acyl-CoAs (for example, stearoyl-CoA) to monounsaturated fatty acyl-CoAs (for example, oleyl-CoA). Given that oleic acids promote the final steps of lipid-rich VLDL assembly and potentiate the secretion of VLDL-TG [49] , we postulate that an inhibition of scd-1 , and the consequent reduction of oleyl-CoA availability and bulk lipid transfer to apoB-lipoproteins in the late stages of their assembly, underlies the MBH oleic acid-induced lowering of hepatic VLDL-TG secretion. Also, it remains a possibility that converging neuronal and hepatic metabolic pathways may mediate the ability of MBH fatty acid sensing to regulate hepatic lipid and glucose homeostasis. These working hypotheses, however, warrant future investigation. Although the specific hypothalamic neuronal population(s) involved in mediating the currently described MBH fatty acid-dependent neurocircuitry remains unknown, our findings implicate a pertinent nutrient-derived approach that functionally stimulates a neural system to modulate metabolism. The involvement of MBH K ATP -channels is of interest since central K ATP -channels also mediate the ability of circulating insulin to retain fatty acids in white adipose tissue in healthy mice [50] . The current study demonstrates that the activation of MBH K ATP -channels, per se , attenuates hepatic VLDL-TG secretion and plasma TG levels in a model of HFD-induced hypertriglyceridemia. Given that orally administered diazoxide, which increased CSF levels of diazoxide and activated brain K ATP -channels in parallel complementary studies in rodents, lowers glucose production in humans [51] , it would be important to assess whether diazoxide lowers VLDL-TG secretion in humans and alternative experimental rodent models with obesity, diabetes and lipid disorders such as the fructose-fed hamster and the apoE-deficient and/or LDLR-deficient mice. Diazoxide inhibits β-cell insulin secretion [52] , and since circulating insulin negatively regulates hepatic VLDL-TG release [14] , systemic diazoxide may not reduce VLDL-TG secretion. To clarify this extrapancreatic role of diazoxide, a pancreatic-euglycemic clamp technique can be utilized to first test the efficacy of activating brain K ATP -channels with systemic diazoxide while maintaining basal plasma insulin levels. This could reveal a lipid-lowering effect of diazoxide that is mediated by brain K ATP -channel activation. In summary, we unveil a fatty acid-dependent hypothalamic–DVC neurocircuitry that regulates hepatic secretion of VLDL-TG and its potential interventional benefit in lowering lipid levels in obesity and diabetes. All experimental protocols in this study were reviewed and approved by the Institutional Animal Care and Use Committee of the UHN. Experimental animals Nine-week-old male SD rats (Charles River Laboratories, Saint-Constant, QC, Canada) weighing 280–300 g were used. Rats were individually housed, subjected to a standard light–dark cycle, and had ad libitum access to drinking water and standard chow (Teklad Global 18% protein, Harlan Laboratories, Madison, WI, USA). Bilateral, 26-gauge, stainless steel guide cannulae (Plastics One Inc, Roanoke, VA, USA) were stereotaxically implanted into the MBH (3.1 mm posterior to bregma, 0.4 mm lateral to midline, 9.6 mm below cranial surface) in anaesthetized (ketamine, 60 mg kg −1 ; xylazine, 8 mg kg −1 ) rats [53] . In one experimental group, bilateral cannulae were also implanted into the DVC (0.4 mm lateral to midline, 7.9 mm below cranial surface, at occipital crest) [27] immediately following MBH cannulation. Indwelling catheters were implanted in the left carotid artery and right jugular vein for blood sampling and infusion 8 days after stereotaxic surgery [27] . Post-surgical body weight and food intake were monitored daily. Rats attained at least 90% of their presurgery body weight before undergoing experimentation. Infusion protocol for VLDL-TG secretion experiments Experiments were performed in 10-h fasted rats 5 days after vascular catheterization. Blood samples were obtained in conscious, unrestrained rats immediately before the start of MBH infusions (0.33 μl per h, CMA 400 syringe pump, CMA Microdialysis, Inc., North Chelmsford, MA) of the following infusates: (i) vehicle (3% cyclodextrin in saline), (ii) oleic acid (1 mmol l −1 , dissolved in vehicle), (iii) rottlerin (60 μmol l −1 ), (iv) oleic acid (1 mmol l −1 )+BIM (60 μmol l −1 ), (v) oleic acid (1 mmol l −1 )+rottlerin (60 μmol l −1 ), (vi) 1-OAG (250 μmol l −1 ), (vii) OAG (250 μmol l −1 )+rottlerin (60 μmol l −1 ), (viii) oleic acid (1 mmol l −1 )+glibenclamide (100 μmol l −1 ), (ix) diazoxide (46.7 μmol l −1 ), (x) diazoxide (46.7 μmol l −1 )+rottlerin (60 μmol l −1 ). Concurrent DVC infusion (0.33 μl per h) in one study consisted of (xi) saline, (xii) MK-801 (0.06 ng min −1 ) or (xiii) glycine (10 μmol l −1 ) with MBH vehicle or MBH oleic acid (1 mmol l −1 ) infusion. These infusate doses were used based on studies involving glucose regulation and/or feeding [28] , [33] , [43] , [54] . Infusions of inhibitors, when used, or saline as a control, commenced at t =−20 min, and infusions of other reagents commenced at t =−10 min and were maintained until the end of the experiment at t =150 min. Time 0-min blood samples were obtained after MBH preinfusions, followed by an intravenous injection of tyloxapol (Sigma-Aldrich, St Louis, MO; 600 mg kg −1 , dissolved in saline, over ~1 min). Blood samples were subsequently obtained every 15 min until t =90 min and every 30 min until the end of the experiment. Plasma was separated by centrifugation and stored at −20 °C until assayed. To prevent hypovolemia and anaemia, packed red blood cells were resuspended in 0.2% heparinized saline and reinfused into the rat. MBH adenovirus injection An adenovirus expressing the DN form of PKC-δ (3.5 × 10 9 p.f.u. ml −1 ; courtesy of Dr J.W. Soh, Incheon, South Korea), or LacZ (3.6 × 10 9 p.f.u. ml −1 ) as a control, was injected into the MBH for one set of experiments [55] . In a separate set of experiments, an adenovirus expressing the DN form of the Kir6.2 subunit of the K ATP -channel (3.1 × 10 10 p.f.u. ml −1 ), or GFP (3.0 × 10 10 p.f.u. ml −1 ) as a control, was injected into the MBH [55] . Adenoviruses were injected (3 μl bilaterally) over 30 s with microsyringes after stereotaxic surgery into the MBH while rats remained under anaesthesia as described [30] , [56] . Eight days after MBH cannulation and adenoviral injection, vascular catheterization was performed. On recovery, virus-injected rats underwent VLDL-TG experiments with MBH oleic acid, OAG, or vehicle infusions as described above. Hepatic branch vagotomy Hepatic branch vagotomy was performed as described [27] . The hepatic branch of the ventral subdiagphragmatic vagal trunk was transected, and the omentum between the liver and oesophagus was severed to remove tissue connections between the liver and oesophagus. Transection of the hepatic vagal nerve disrupts neural communication between the CNS and liver. Sham operation consisted of the same procedure except for transection of the hepatic vagal nerve. After a 5-day recovery, rats underwent VLDL-TG experiments with MBH oleic acid or vehicle infusions as explained above. High-fat feeding Another group of rats were fed a palatable, lard oil enriched, HFD (TestDiet #57IR, Purina Mills, Richmond, IN) for 3 days. HFD had greater total calorie content, greater fat content (33 versus 17%) and less protein (22 versus 31%) and carbohydrate content (45 versus 52%). Two days after vascular catheterization, regular chow was replaced with HFD and food intake was measured for 3 days of HFD feeding leading to the experimental day. Rats that did not overeat were excluded from the study. Rats were similarly subjected to a 10-h fast on the night before the VLDL-TG secretion experiment with MBH oleic acid, OAG, diazoxide or vehicle infusions as described above. In a separate group of rats, hepatic vagotomy or sham operation was performed as described above immediately preceding vascular catheterization, and HFD was subsequently given as indicated. Plasma metabolites and hormones analyses Plasma TG (Roche Diagnostics, Indianapolis, IN), FFA (Wako Diagnostics, Richmond, VI), insulin, leptin, adiponectin (RIA; Linco Research Inc., St Charles, MO/Millipore Corporation, Billerica, MA), HDL cholesterol and LDL/VLDL cholesterol (Abcam Inc., Toronto, ON) and total bile acid (Crystal Chem, Inc., Downers Grove, IL) levels were measured using commercial kits. Plasma glucose was measured with a glucose analyser using the glucose oxidase method (GM9, Analox Instruments, Lunenburg, MA). Plasma apoB analysis ApoB measurements were performed as described [27] . In brief, t =0 and t =150 plasma samples from rats that underwent tyloxapol experiments were diluted 50 × in distilled water before being prepared for SDS–polyacrylamide gel electrophoresis. Each lane contained 5 μl of denatured plasma. Samples were resolved using a 4–15% gradient polyacrylamide gel and detected using chemiluminescent immunoblotting using a commercial apoB antibody (1/100 dilution; sc-11795 goat, Santa Cruz Biotechnology, Inc., Dallas, TX). Western blots were performed as below. PKC-δ translocation assay The plasma membrane translocation of MBH PKC-δ was evaluated by measuring protein levels in cytosolic and plasma membrane fractions. MBH tissue wedges from rats that received MBH infusions of oleic acid (1 mmol l −1 ) or OAG (250 μmol l −1 ) or vehicle (3% cyclodextrin in saline) for 5 min were collected and immediately frozen. Cytosolic and plasma membrane protein fractions were isolated using a commercial kit suitable for mammalian tissues (Plasma Membrane Protein Extraction Kit #K268-50, BioVision Incorporated, Milpitas, CA). Cytosolic and purified plasma membrane fraction protein concentrations were measured using a BCA Protein Assay kit (#K812-1000, BioVision Incorporated, Milpitas, CA) and 4 μg of protein was subjected to electrophoresis on 9% polyacrylamide gels and transferred to nitrocellulose membranes. Conditions of blocking and incubation of primary and secondary antibodies are described below. Immunoblots were detected on films processed with a SRX-101A film developer (Konica Minolta Medical Imaging USA, Inc., Wayne, NJ), scanned with a GS-800 Calibrated Densitometer (Bio-Rad Laboratories, Mississauga, ON, Canada) and quantified with ImageJ software. Primary antibodies diluted 1/1,000 with 5% bovine serum albumin (BSA) in TBS-T included: PKC-δ (sc-213 rabbit, Santa Cruz); IL β (L55B10 mouse, #3020, Cell Signaling Technology, Danvers, MA); and MEK1/2 (L38C12 mouse, #4694, Cell Signaling). Liver biochemical analyses Liver tissue from rats that underwent tyloxapol experiments were collected and immediately frozen for hepatic protein, mRNA and TG measurements as described below. Western blot analyses Liver and MBH were homogenized as described [53] . Liver and MBH were homogenized in lysis buffer containing 50 mM Tris-HCl (pH 7.5), 1 mM EGTA, 1 mM EDTA, 1% (w/v) Non-idet P40, 1 mM sodium orthovanadate, 50 mM sodium fluoride, 5 mM sodium pyrophosphate, 0.27 M sucrose, 1 mM DTT, and protease inhibitor cocktail EDTA-free (Roche Diagnostics). The homogenate was centrifuged at 14,000 g for 5 min at 4 °C, and protein concentration of the supernatant was determined using Pierce’s 660 nm Protein Assay. Liver (40 μg) and MBH (10 μg) total protein lysates were subjected to electrophoresis using polyacrylamide gels and transferred to nitrocellulose membranes. Membranes were incubated with blocking solution (5% BSA in Tris-buffered saline containing 0.2% Tween-20 (TBS-T)) for 1 h at room temperature and overnight at 4 °C in primary antibody solutions as indicated below. Protein expression was detected using an HRP-linked secondary antibody (diluted 1/4,000 in blocking solution) and an enhanced chemoluminescence reagent (Pierce ECL Western Blotting Substrate, Thermo Scientific, Rockford, IL). Immunoblots were detected using a MicroChemi 4.2 chemiluminescent imaging system and quantified with GelQuant image analysis software (DNR Bio-Imaging Systems, Jerusalem, Israel). Primary antibodies diluted as indicated with 5% BSA in TBS-T included: phosphorylated and total ACC (1/1,000; #3661, #3676 rabbit, Cell Signaling), FAS (1/1,000; 610962 human, BD Biosciences, Mississauga, ON), DGAT1 (1/2,000) and DGAT2 (1/1,000) (NB110-41487, NBP1-71700 rabbit, Novus Biologicals Canada ULC, Oakville, ON), MTP (1/5,000; 612022 mouse, BD Biosciences), PKC-δ (sc-213 rabbit, Santa Cruz) and PKC-ε (sc-214 rabbit, Santa Cruz). See Supplementary Fig. 4 for uncropped blots. Hepatic gene expression analyses Hepatic RNA extraction (using a commercially available kit (PureLink RNA Mini Kit, Ambion) and quantitative real-time PCR were performed as previously described [53] . Quantitative real-time PCR was performed (ABI Prism 7900) using TaqMan Gene Expression Assays (sdc-1 ( Scd-1 , Rn00594894_g1); srebp-1 ( Srebf1 , Rn01495769_m1); pparα ( Ppara , Rn00566193_m1); pparγ ( Pparg , Rn00440945_m1); and ribosomal protein 18s ( Rps18 , Rn01428915_g1)) and TaqMan Gene Expression Master Mix (Applied Biosystems). Expression values were normalized to the internal control gene, 18 s, for the efficiency of amplification and quantified by the 2 −ΔΔ C t method [57] . Hepatic TG extraction Triglycerides were extracted using a chloroform:methanol procedure before proceeding to TG assay as described above. Statistical analyses Unpaired, two-tailed t -tests were used for the statistical analyses of two groups. ANOVA was performed where comparisons were made across more than two groups, and if significant, a Dunnett’s post hoc test was used to allow the comparisons of treatments to a single group. Repeated measures ANOVA was performed to compare measurements taken repeatedly over time, and if significant, a Duncan’s post hoc test was used to determine the statistical significance between groups. Unless otherwise stated, significance was deemed when P <0.05. Sample sizes for groups presented in Figures are indicated in the figure legends or otherwise indicated in Results. Data are presented as mean±s.e.m. unless stated otherwise. How to cite this article : Yue, J. T. Y. et al . A fatty acid-dependent hypothalamic–DVC neurocircuitry that regulates hepatic secretion of triglyceride-rich lipoproteins. Nat. Commun. 6:5970 doi: 10.1038/ncomms6970 (2015).